Catalytic asymmetric dearomatization of phenols via divergent intermolecular (3 + 2) and alkylation reactions The catalytic asymmetric dearomatization (CADA) reaction has proved to be a powerful protocol for rapid assembly of valuable three-dimensional cyclic compounds from readily available planar aromatics. In contrast to the well-studied indoles and naphthols, phenols have been considered challenging substrates for intermolecular CADA reactions due to the combination of strong aromaticity and potential regioselectivity issue over the multiple nucleophilic sites (O, C2 as well as C4). Reported herein are the chiral phosphoric acid-catalyzed divergent intermolecular CADA reactions of common phenols with azoalkenes, which deliver the tetrahydroindolone and cyclohexadienone products bearing an all-carbon quaternary stereogenic center in good yields with excellent ee values. Notably, simply adjusting the reaction temperature leads to the chemo-divergent intermolecular (3 + 2) and alkylation dearomatization reactions. Moreover, the stereo-divergent synthesis of four possible stereoisomers in a kind has been achieved via changing the sequence of catalyst enantiomers. The catalytic asymmetric dearomatization (CADA) reaction is a powerful transformation for directly converting planar aromatic compounds into enantioenriched three-dimensional cyclic scaffolds. Over the past decades, significant progress in this field has been made by You and others, which largely contributed to the facile synthesis of natural products and biologically important molecules [1] , [2] , [3] , [4] , [5] . For example, indole derivatives have been utilized frequently as model substrates for CADA reactions due to their relatively weak aromaticity [6] , [7] , [8] , [9] , [10] . Naphthols can be treated as conjugated enols in a sense, undergoing CADA transformations to prepare partially dearomatized naphthalenones [11] , [12] , [13] , [14] , [15] . On the other hand, the CADA reaction of phenols, readily available chemical feedstocks, still remains elusive (Fig. 1A ). Oxidative asymmetric dearomatization of substituted phenols can be achieved by using oxidation systems as exampled by the chiral hypervalent iodine/ m -CPBA [16] , [17] , [18] . Alternatively, the combination of oxidative dearomatization and subsequent asymmetric desymmetrization has been employed conventionally as a stepwise strategy for the asymmetric dearomatization of phenols (Fig. 1B ) [19] , [20] , [21] . Direct non-oxidative asymmetric dearomatization of phenols is considered challenging, since the regioselectivity issue over the multiple nucleophilic sites (O, C2 as well as C4) is problematic. As such, phenol substrates are often delicately designed by incorporating an electrophilic group to conduct intramolecular dearomative cyclizations (Fig. 1C ). For instance, metal-catalyzed intramolecular para -position allylation [22] , [23] , arylation [24] , [25] , [26] , [27] , and alkylation [28] were disclosed by You, Tang and others. Recently, intramolecular ortho -position asymmetric dearomatization reactions of phenols have been reported by Ye and others via activation of ynamides or alkynes [29] , [30] . In a sharp contrast, intermolecular CADA reactions of common phenols, especially the cycloaddition reactions, are far less developed [31] . Fig. 1: Asymmetric dearomatization of phenols. A Aromatics in CADA; B stepwise strategy; C intramolecular strategy; D intermolecular (3 + 2) and alkylation reactions (this work). Full size image Given the potential regio-, chemo-, and stereo-selectivity issues associated in the intermolecular CADA reaction of phenols, the rational selection of catalytic system and electrophile is key to success. Azoalkenes have emerged as versatile synthons in asymmetric synthesis, as they allow the rapid assembly of valuable N-heterocycles [32] , [33] . For instance, in situ generated azoalkenes have been employed as four-atom building blocks in copper-catalyzed (4 + n ) reactions by Wang and others [34] , [35] , [36] , [37] , [38] , [39] . Recently, we have found that existent azoalkenes could act as three-atom synthons in chiral phosphoric acid (CPA)-catalyzed reacitons [40] , [41] , [42] , [43] . Along this line, we report herein the intermolecular CADA reaction of common phenols 1 with azoalkenes 2 under the catalysis of CPA (Fig. 1D ). Notably, this protocol is featured by the temperature-dependent chemo-divergence and the sequence-dependent stereo-divergence [44] . By simply adjusting the reaction temperature, the chemo-divergent intermolecular (3 + 2) and alkylation dearomatization reactions of phenols have been accomplished, which deliver the corresponding products 3 and 4 bearing an all-carbon quaternary stereogenic center in good yields with excellent ee values. Meanwhile, with only a single CPA catalyst, changing the use sequence of catalyst enantiomers results in the stereo-divergent synthesis of four possible stereoisomers in a kind. Additionally, the constructed bicyclic tetrahydroindolone bearing an all-carbon quaternary stereogenic center is the core structure of some bioactive natural alkaloids, such as mesembrine, crinine and powelline [45] , [46] , [47] , [48] , [49] . 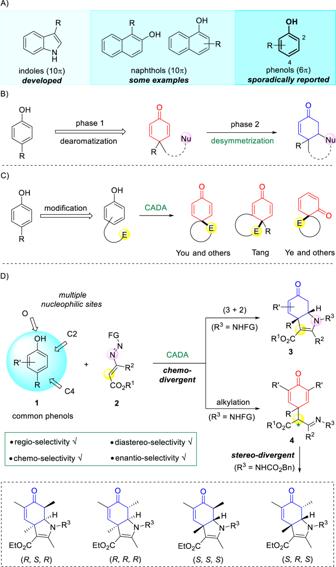Fig. 1: Asymmetric dearomatization of phenols. AAromatics in CADA;Bstepwise strategy;Cintramolecular strategy;Dintermolecular (3 + 2) and alkylation reactions (this work). We commenced our investigation with the model reaction between p -cresol 1a and azoalkene 2a (Table 1 ). In view of the potential regio- and chemo-selectivity issues, 3a–6a could be the products. Firstly, Brønsted acids were employed. Under the catalysis of CPA-1 in toluene at 25 °C, intermolecular CADA reaction occurred, delivering the only (3 + 2) product 3a in a good yield with a moderate enantioselectivity (entry 1). Then, a series of CPAs were screened to find the optimal catalyst. While all the binol-derived CPAs failed to improve the ee value (entries 2−6), spinol-derived CPA-7 gave an encouraging result wherein the ee value was increased to a relatively higher level (entry 7). So, CPA-7 was selected as the best catalyst for the subsequent condition screening. Solvent effect was studied, indicating that toluene was the best choice (entry 7 vs 8–10). Lowering reaction temperature contributed to the enantio-control (entries 11−12). Finally, additives were used to further optimize the reaction. With 5 Å molecular sieve, both the yield and ee value of product 3a could be improved to a high level (entry 14). Interestingly, Lewis acids led to a different regioselective result (see Supplementary Information for details). For example, while AgOTf offered the (3 + 2) dearomatization product 3a (entry 16), AgOAc resulted in the oxa -Michael addition product 5a (entry 15). We tried to control enantioselectivity of this oxa -Michael process by using silver chiral phosphate. However, only dearomative (3 + 2) product 3a was obtained (entry 17), which indicated silver chiral phosphate could also catalyze the dearomatization process. Notably, none of the C4-dearomatization alkylation product 4a and C2-Friedel-Crafts alkylation product 6a were observed during the optimization. Table 1 Reaction optimization a Full size table With the best reaction conditions in hand, the reaction generality of azoalkenes was examined. As shown in Fig. 2 , the reaction was applicable to a variety of azoalkenes. The N -protective group could be varied from -CO 2 Bn ( 3a ) to -CO 2 Me ( 3b ), -CO 2 Et ( 3c ), and -CO 2 fluorenylmethyl ( 3d ) with consistently excellent ee values. The ester moiety appended to the C=C double bond had little effect on the reaction efficiency, all the tested substrates ( 3e−3j ) were well-tolerated. In contrast, the R 2 group significantly affected the enantioselectivity of the reaction. The larger the R 2 group, the lower the ee values ( 3k−3l ).Next, we turned our attention to the substrate scope of phenols (Fig. 2 ). Various phenols bearing alkyl substituents at 4-position, such as ethyl ( 3m ), n propyl ( 3n ), n butyl ( 3o ) and n pentyl ( 3p ) groups as well as allyl group ( 3q ), served as suitable substrates for this CADA (3 + 2) reaction, allowing the installation of different moieties at the quaternary stereogenic center. In addition, the hindered cyclopropyl group ( 3r ) worked equally well under standard conditions. Notably, the aryl group at the 4-position was also tolerated, as product 3s was readily prepared. Furthermore, we examined the tolerance of the reaction to di-substituted phenols. Products 3t−3z were prepared in good yields with good to excellent enantioselectivities under the modified conditions. Among them, the alkyl groups at the C2-position were in favor of enantio-control ( 3t−3v ), while methoxy group resulted in a slight decrease in ee value ( 3w ). Substituents at the C3-position had some delicate influence on the reaction. For example, 3x and 3y were obtained in good ee values, while 3z was formed in an excellent enantioselectivity. A regio-isomer was observed in the preparation of 3x (see Supplementary Information for details). Remarkably, the projected reaction was applicable to 1-naphthol, leading to the corresponding product 3a’ in good yield and ee value. The absolute configurations of the products were assigned based on X-ray crystallographic analysis of 3t . Fig. 2: Substrate scope for CADA (3 + 2) reaction. Reaction conditions: 1 (0.2 mmol), 2 (0.24 mmol. ), CPA-7 (10 mol%), and 5 Å MS (50 mg) in toluene (1 mL) at –30 °C for 12 h, isolated yields, ee and dr values were determined by chiral HPLC analysis, all dr >20:1, PG = NHCO 2 Bn. a with 3 Å MS (50 mg) and CPA-2 at −40 °C. b with 3 Å MS (50 mg) and CPA-4 at 25 °C. Full size image Encouraged by the success of CADA (3 + 2) reaction of mono- and di-substituted phenols, we then studied the substrate scop by employing tri-substituted phenols. Unexpectedly, the temperature-dependent chemo-divergent dearomatization reactions of phenol 1o were observed (Fig. 3A ). At –30 °C, the standard conditions delivered the only dearomative alkylation product 4b in an excellent yield and with an excellent ee value. On the other hand, the CADA (3 + 2) reaction product 8 was obtained at 25 °C. Given the synthetic and biological importance of chiral cyclohexadienones, the substrate scope of this intermolecular catalytic asymmetric alkylation dearomatization had been studied (Fig. 3B ). The examination of various azoalkenes indicated that the R 2 group had some influence on the reaction efficiency. Reactions using methyl substituted azoalkenes (R 2 = Me) were conducted smoothly, affording the corresponding cyclohexadienone products 4c–4i in good yields with excellent enantioselectivities (76–93% yields, 96–>99% ee ). However, the steric hindered ethyl ( 4j ), n butyl ( 4k ), and benzyl ( 4l ) groups were not well compatible, which was same as the (3 + 2) process. The generality of tri-substituted phenols was also investigated. While electron-donating methoxy group ( 4m ) afforded the consistently good yield and ee value, electron-withdrawing bromo group ( 4n ) gave the result of no reaction. Fig. 3: Chemo-divergent (3 + 2) and alkylation dearomatization reactions. A Reaction discovery; B substrate scope. Reaction conditions: 1 (0.2 mmol), 2 (0.24 mmol. ), CPA-7 (10 mol%), and 3 Å MS (50 mg) in toluene (1 mL) at −30 °C for 12 h, isolated yields, ee value was determined by chiral HPLC analysis. Full size image To gain insights into the reaction mechanism, some control experiments were performed (Fig. 4 ). Firstly, enantioenriched 4b was subjected to the standard conditions at room temperature. Product 8 was formed in an excellent yield and with good stereoselectivities (Fig. 4A ), which clearly suggested that 8 is a productive intermediate for the (3 + 2) reaction. More importantly, with the same enantioenriched 4b , ( S )- CPA-7 led to a different diastereoisomer 9 (Fig. 4B ), which implied the substrate control for the enantioselectivity and catalyst control for the diastereoselectivity. These results paved the way to a sequence-dependent stereo-divergent synthesis enabled by one chiral catalyst. Namely, changing the use sequence of ( R )- CPA-7 and ( S )- CPA-7 could result in the stereo-divergent synthesis of four possible stereoisomers in a kind. To demonstrate this concept, four possible stereoisomers of the (3 + 2) reaction products were prepared from 1o and 2a (Fig. 4E ). However, under the catalysis of (±)- CPA-7 , racemization of 4b was observed which led to a low ee value of the cyclizaiton product (Fig. 4C ). On the other hand, when racemic 4b was employed, the enantio-convergent desymmetrization of cyclohexadienone was achieved (Fig. 4D ), which will be fully investigated in the future. Based on these experimental results, a plausible reaction pathway and possible transition states ( TS ) were suggested in Fig. 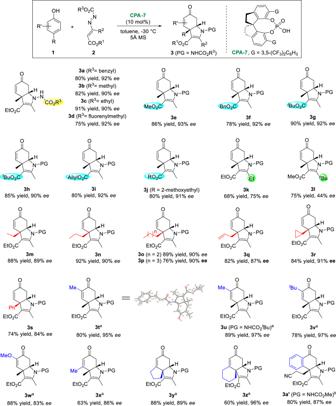Fig. 2: Substrate scope for CADA (3 + 2) reaction. Reaction conditions:1(0.2 mmol),2(0.24 mmol.),CPA-7(10 mol%), and 5 Å MS (50 mg) in toluene (1 mL) at –30 °C for 12 h, isolated yields,eeand dr values were determined by chiral HPLC analysis, all dr >20:1, PG = NHCO2Bn.awith 3 Å MS (50 mg) andCPA-2at −40 °C.bwith 3 Å MS (50 mg) andCPA-4at 25 °C. 4F . In TS-1, CPA-7 simultaneously activated phenol 1a and azoalkene 2a via dual hydrogen-bonding interactions. The CPA-catalyzed asymmetric dearomative alkylation of phenol 1a with azoalkene 2a occurred, generating the hydrazone intermediate Int-1 with a chiral carbon center. Subsequently, the group selectivity was accomplished via substrate-controlled enantioselective intramolecular cyclization. While pathway a led to the unfavored iminium Int-2 due to the sterically hindered cis -orientation of methyl and ester groups, pathway b gave the favored one Int-3 . The final CPA-catalyzed diastereoselective proton transfer via tautomerization facilitated the (3 + 2) process and delivered the dearomative product 3a . Fig. 4: Mechanistic considerations and stereo-divergent synthesis. A Cyclization of enantioenriched 4b with ( R )- CPA-7 ; B cyclization of enantioenriched 4b with ( S )- CPA-7 ; C cyclization of enantioenriched 4b with racemic CPA-7 ; D Cyclization of racemic 4b with ( R )- CPA-7 ; E stereo-divergent synthesis; F proposed reaction pathway and transition states. Full size image Finally, to examine the practicality of this protocol, a convenient gram-scale synthesis of 3u was conducted under standard reaction conditions (see Supplementary Information for details). Then a series of derivatizations were performed, further highlighting the synthetic utility (Fig. 5 ). Firstly, the enone motif could be manipulated via 1,2-addition, 1,4-hydrogenation and 1,2-reduction affording the corresponding product 10 – 12 in good yields and without erosion of enantiomeric purity. Besides, the protecting group on the azo nitrogen center could be easily removed, yielding product 13 in a good yield of 93%. Notably, N -allylic alkylation of 3a led to the formation of compound 14 incorporating a N−N axially stereogenic axis. The N−N bond cleavage had been achieved via a base-promoted eliminative strategy, furnishing the amine product 15 . Fig. 5: Preliminary applications. Reaction conditions: i) 3c (0.2 mmol), CH 3 MgBr (0.3 mmol. ), THF, 0 °C; ii) 3c (0.3 mmol), Pd/C, H 2 , MeOH, r.t.; iii) 3u (0.2 mmol), NaBH 4 (0.2 mmol), MeOH, 0 °C; iv) 3 u (0.2 mmol), TFA (0.2 mL), CH 2 Cl 2 , 0 °C; v) 3a (0.2 mmol), ethyl 2-bromoacetate (0.24 mmol), Cs 2 CO 3 (0.3 mmol), CH 3 CN, r.t.; vi) 3u (0.2 mmol), ethyl 2-bromoacetate (0.24 mmol), Cs 2 CO 3 (0.3 mmol), CH 3 CN, r.t. then reflux. Full size image In conclusion, we have established the CPA-catalyzed divergent intermolecular CADA reactions of common phenols with azoalkenes, which deliver the tetrahydroindolone and cyclohexadienone products bearing an all-carbon quaternary stereogenic center in good yields with excellent ee values. As opposite to the previous dearomatization reactions involving indoles and naphthols, this work employs readily available phenols, which have been considered challenging substrates for intermolecular asymmetric dearomatization reactions due to the combination of strong aromaticity and the potential regioselectivity issue over the multiple nucleophilic sites (O, C2 as well as C4). Notably, this reaction is featured by the temperature-dependent chemo-divergence and the sequence-dependent stereo-divergence. Simply adjusting the reaction temperature leads to the chemo-divergent intermolecular (3 + 2) and alkylation dearomatization reactions. More importantly, stereo-divergent synthesis of four possible stereoisomers in a kind has been achieved by changing the sequence of catalyst enantiomers. Further applications of this protocol are currently ongoing in our laboratory and will be reported in due course. Typical procedure for (3 + 2) reaction Para substituted phenols 1 (0.20 mmol), 5 Å MS (50 mg), ( R )-CPA-7 (10 mol%) were dissolved in toluene (1 mL), and azoalkenes 2 (0.24 mmol) were added dropwise at −30 °C. The reaction mixture was stirred at the same temperature for 12 h. The solvent was removed in vacuo and the crude product was separated by flash column chromatography on silica gel (petroleum ether/ethyl acetate 3:1–1:1) to afford the products 3 . Typical procedure for alkylation reaction Tri-substituted phenols 1 (0.20 mmol), 3 Å MS (50 mg) and ( R )-CPA-7 (10 mol%) were dissolved in toluene (1 mL), and azoalkenes 2 (0.24 mmol) were added dropwise at –30 °C. 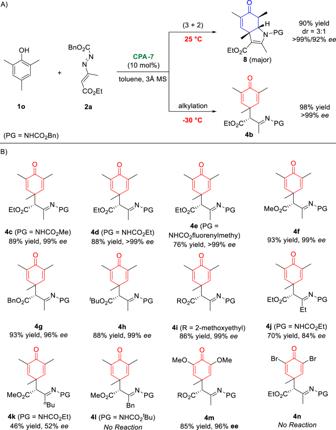Fig. 3: Chemo-divergent (3 + 2) and alkylation dearomatization reactions. AReaction discovery;Bsubstrate scope. Reaction conditions:1(0.2 mmol),2(0.24 mmol.),CPA-7(10 mol%), and 3 Å MS (50 mg) in toluene (1 mL) at −30 °C for 12 h, isolated yields,eevalue was determined by chiral HPLC analysis. 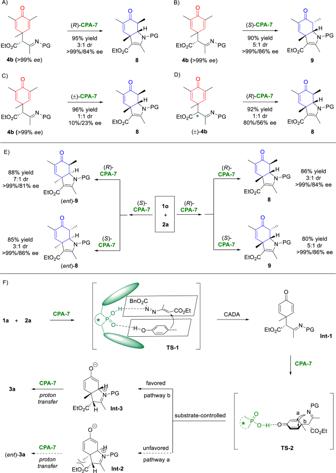Fig. 4: Mechanistic considerations and stereo-divergent synthesis. ACyclization of enantioenriched4bwith (R)-CPA-7;Bcyclization of enantioenriched4bwith (S)-CPA-7;Ccyclization of enantioenriched4bwith racemicCPA-7;DCyclization of racemic4bwith (R)-CPA-7;Estereo-divergent synthesis;Fproposed reaction pathway and transition states. 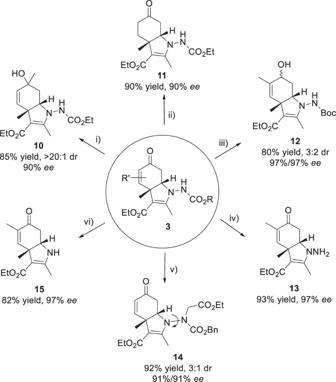Fig. 5: Preliminary applications. Reaction conditions: i)3c(0.2 mmol), CH3MgBr (0.3 mmol.), THF, 0 °C; ii)3c(0.3 mmol), Pd/C, H2, MeOH, r.t.; iii)3u(0.2 mmol), NaBH4(0.2 mmol), MeOH, 0 °C; iv)3u(0.2 mmol), TFA (0.2 mL), CH2Cl2, 0 °C; v)3a(0.2 mmol), ethyl 2-bromoacetate (0.24 mmol), Cs2CO3(0.3 mmol), CH3CN, r.t.; vi)3u(0.2 mmol), ethyl 2-bromoacetate (0.24 mmol), Cs2CO3(0.3 mmol), CH3CN, r.t. then reflux. The reaction mixture was stirred for 12 h. The solvent was removed in vacuo and the crude product was separated by flash column chromatography on silica gel (petroleum ether/ethyl acetate 3:1–1:1) to afford the products 4 .